Conformational landscapes of DNA polymerase I and mutator derivatives establish fidelity checkpoints for nucleotide insertion The fidelity of DNA polymerases depends on conformational changes that promote the rejection of incorrect nucleotides before phosphoryl transfer. Here, we combine single-molecule FRET with the use of DNA polymerase I and various fidelity mutants to highlight mechanisms by which active-site side chains influence the conformational transitions and free-energy landscape that underlie fidelity decisions in DNA synthesis. Ternary complexes of high fidelity derivatives with complementary dNTPs adopt mainly a fully closed conformation, whereas a conformation with a FRET value between those of open and closed is sparsely populated. This intermediate-FRET state, which we attribute to a partially closed conformation, is also predominant in ternary complexes with incorrect nucleotides and, strikingly, in most ternary complexes of low-fidelity derivatives for both correct and incorrect nucleotides. The mutator phenotype of the low-fidelity derivatives correlates well with reduced affinity for complementary dNTPs and highlights the partially closed conformation as a primary checkpoint for nucleotide selection. The remarkable fidelity of DNA synthesis is crucial for genome stability [1] . This fidelity depends on non-covalent transitions preceding the chemical step of phosphoryl transfer and serving as checkpoints whereby inappropriate substrates are rejected early during the reaction [2] . Among these transitions, the fingers-closing transition is of particular interest: the binding of the complementary dNTP to a polymerase-DNA (Pol-DNA) binary complex leads to a conformational change in which a part of the fingers subdomain (including the O-helix) moves from an open to a closed conformation ( Fig. 1a–c ), and forms a tight binding pocket around the nascent base pair [3] , [4] , [5] , [6] . Previously, we used single-molecule fluorescence resonance energy transfer (FRET) to examine fingers-closing in the Escherichia coli DNA polymerase I (Klenow fragment) (KF; see Santoso et al . [7] ). Our results identified the open and closed conformations that predominate in the binary Pol-DNA and ternary Pol-DNA-dNTP (complementary) complexes, respectively, and showed that the unliganded polymerase explores both open and closed conformations [7] , [8] , [9] , [10] . We also showed that ternary complexes with non-complementary dNTPs or complementary ribonucleotides form distinct FRET species (with FRET signals intermediate between the open and closed states). 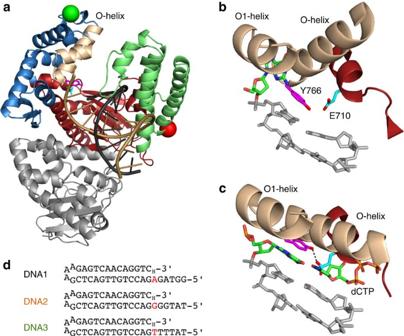Figure 1: Structural view of DNA polymerase I and key residues in this study. (a) The open Pol-DNA binary complex (PDB accession code1L3U) is illustrated using structural data fromBacillus stearothermophilus(Bst) DNA polymerase4, a close homologue of KF. In the following, the KF numbering scheme is used. The fingers subdomain is coloured blue with the exception of the O- and O1-helices coloured beige, the thumb green, the palm subdomain red and the 3'–5' exonuclease grey. The DNA template strand is coloured brown and the DNA primer strand black. The amino acid Y766 is coloured magenta and E710 cyan. The positions of the residues used for labelling are shown as a red sphere for the acceptor (residue 550) and a green sphere for the donor (residue 744). See alsoSupplementary MethodsandSupplementary Table S1for details regarding site-specific labelling. (b) Position of E710 and Y766 in the Pol-DNA binary complex (PDB accession code1L3U). The O-helix is in the open conformation, Y766 is stacked on the template base of the terminal base pair and the next templating base is in a pocket between the O- (mobile) and O1- (immobile) helices. The last two base pairs of the template-primer duplex are in grey. (c) Position of E710 and Y766 in the Pol-DNA-dNTP (correct) ternary complex (PDB accession code1LV5(ref.4)). With the O-helix in the closed position, Y766 has moved away from the terminal base pair, creating space for the templating base. Y766 forms a hydrogen bond with E710, shown as dashed black line. (d) DNA oligonucleotides used in this study. A dideoxy nucleotide (3'-H) prevents extension of the 3' terminus. The templating base is shown in red. Figure 1: Structural view of DNA polymerase I and key residues in this study. ( a ) The open Pol-DNA binary complex (PDB accession code 1L3U ) is illustrated using structural data from Bacillus stearothermophilus (Bst) DNA polymerase [4] , a close homologue of KF. In the following, the KF numbering scheme is used. The fingers subdomain is coloured blue with the exception of the O- and O1-helices coloured beige, the thumb green, the palm subdomain red and the 3'–5' exonuclease grey. The DNA template strand is coloured brown and the DNA primer strand black. The amino acid Y766 is coloured magenta and E710 cyan. The positions of the residues used for labelling are shown as a red sphere for the acceptor (residue 550) and a green sphere for the donor (residue 744). See also Supplementary Methods and Supplementary Table S1 for details regarding site-specific labelling. ( b ) Position of E710 and Y766 in the Pol-DNA binary complex (PDB accession code 1L3U ). The O-helix is in the open conformation, Y766 is stacked on the template base of the terminal base pair and the next templating base is in a pocket between the O- (mobile) and O1- (immobile) helices. The last two base pairs of the template-primer duplex are in grey. ( c ) Position of E710 and Y766 in the Pol-DNA-dNTP (correct) ternary complex (PDB accession code 1LV5 (ref. 4 )). With the O-helix in the closed position, Y766 has moved away from the terminal base pair, creating space for the templating base. Y766 forms a hydrogen bond with E710, shown as dashed black line. ( d ) DNA oligonucleotides used in this study. A dideoxy nucleotide (3'-H) prevents extension of the 3' terminus. The templating base is shown in red. Full size image The fidelity and speed of DNA replication can be profoundly affected by substitution of amino acids near the polymerase active site [11] , [12] , [13] , [14] , implying that specific side chains control the discrimination between correct and incorrect nucleotides. Two well-studied amino acids contributing to fidelity in KF are E710 and Y766 ( Fig. 1a ), both universally conserved within A-family polymerases [15] . Residue E710 helps in positioning the incoming nucleotide by interacting with the dNTP base-sugar portion, and acts as a steric gate that blocks incorporation of ribonucleotides [16] . Residue Y766 stacks on the template base of the terminal base pair and blocks the insertion site in the binary complex ( Fig. 1b ). Upon fingers-closing, Y766 rotates away from the terminal base pair and is replaced by the templating base, which moves into the catalytic pocket ( Fig. 1c ); the hydrogen-bonded Y766-E710 pair creates part of the binding pocket and controls the nascent base-pair geometry. Here, we report a conformational analysis of wild-type KF (wt KF) and KF derivatives with single amino-acid substitutions at E710 and Y766, respectively, and obtain conformational energy landscapes for various complexes along the prechemistry pathway. Three of the substitutions examined (E710A, Y766A and E710Q) decrease fidelity, acting as ‘mutators’ [11] , [12] , [13] , [14] ; we also analysed Y766F, a derivative with enzymatic properties similar to wt KF [11] , [14] . Since mutators fail to transition efficiently from the partially closed to the closed conformation, our results indicate that the partially closed state is an important fidelity checkpoint and that residues E710 and Y766 are essential for the discrimination between complementary and non-complementary nucleotides. wt KF shows an on-pathway intermediate The conformational profiles for wt KF alone and in complexes with non-extendable DNA substrates ( Fig. 1d ) are shown in Fig. 2a . The unliganded polymerase exhibits a broad FRET distribution ( Fig. 2a , row 1), slightly biased towards an open conformation (60% occupancy, E* lowFRET ~0.48). Formation of the KF–DNA binary complex (using DNA1, Fig. 1d ) further increases the open-state occupancy (81%, E* open ~0.45; Fig. 2a , row 2). The peak positions of the low-FRET species are slightly different in the unliganded polymerase and the binary complex; this is mainly because of unliganded polymerase dynamics [7] , [8] , [10] , but may also be due to conformational states other than the open and closed states, as discussed below. 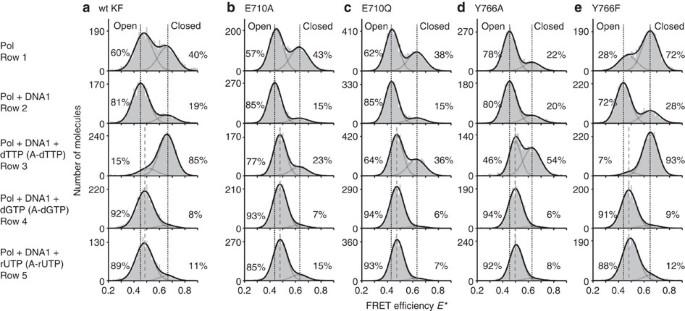Figure 2: Conformational profiles for wt KF and its derivatives. Histograms of the FRET efficiencyE*for wt KF (a), E710A (b), E710Q (c), Y766A (d)and Y766F (e). Each histogram (70 bins) was derived from several thousand fluorescence bursts detected from labelled polymerases diffusing through a confocal spot. The histograms were fitted to a double-Gaussian model to determine the relative occupancies (shown as percentages) and mean peak positions of the individual FRET species (black lines, sum of Gaussians; grey lines, individual Gaussians). First row: unliganded polymerase (Pol). Second row: binary complex, formed by adding DNA1 (with A as the templating base, final DNA concentration: 100 nM) to the polymerase (Pol+DNA). Third row: ternary complex with the correct nucleotide, formed by adding dTTP (1 mM) to the binary complex. Fourth row: ternary complexes with an incorrect nucleotide, formed by adding dGTP (1 mM) to the binary complex. Fifth row: ternary complex with the complementary ribonucleotide, formed by adding rUTP (1 mM) to the binary complex. The two dotted vertical lines mark the meanE*values of the open and closed FRET species in the binary complex. Histograms for each enzyme were measured on the same day. The dashed line marks the meanE*value of the intermediate-FRET species as populated in the ternary complexes (see alsoSupplementary Fig. S1). Figure 2: Conformational profiles for wt KF and its derivatives. Histograms of the FRET efficiency E* for wt KF ( a ), E710A ( b ), E710Q ( c ), Y766A ( d) and Y766F ( e ). Each histogram (70 bins) was derived from several thousand fluorescence bursts detected from labelled polymerases diffusing through a confocal spot. The histograms were fitted to a double-Gaussian model to determine the relative occupancies (shown as percentages) and mean peak positions of the individual FRET species (black lines, sum of Gaussians; grey lines, individual Gaussians). First row: unliganded polymerase (Pol). Second row: binary complex, formed by adding DNA1 (with A as the templating base, final DNA concentration: 100 nM) to the polymerase (Pol+DNA). Third row: ternary complex with the correct nucleotide, formed by adding dTTP (1 mM) to the binary complex. Fourth row: ternary complexes with an incorrect nucleotide, formed by adding dGTP (1 mM) to the binary complex. Fifth row: ternary complex with the complementary ribonucleotide, formed by adding rUTP (1 mM) to the binary complex. The two dotted vertical lines mark the mean E* values of the open and closed FRET species in the binary complex. Histograms for each enzyme were measured on the same day. The dashed line marks the mean E* value of the intermediate-FRET species as populated in the ternary complexes (see also Supplementary Fig. S1 ). Full size image Addition of the complementary nucleotide (A-dTTP) forms a ternary complex, wherein ~85% of all molecules display a closed conformation ( E* closed ~0.66; Fig. 2a , row 3). Notably, the presence of 1 mM dTTP (instead of 10 μM used previously [7] ) increases significantly the E* of the low-FRET species ( E* lowFRET ~0.51) compared with the E* open in the binary complex (see Supplementary Fig. S1 ). Indeed, the E* lowFRET for 1 mM dTTP is closer to the intermediate-FRET species ( E* ~0.48) also populated by complexes containing 1 mM of either non-complementary dNTP or complementary rNTP (A-dGTP and A-rUTP, respectively; Fig. 2a , rows 4 and 5). For both A-dGTP and A-rUTP ternary complexes, the occupancy ratio of the E* ~0.48 FRET species and the closed conformation is ~9:1. We measured nucleotide-binding affinities by analysing FRET histograms generated at different nucleotide concentrations ( Fig. 3a ). The equilibria between the FRET species are depicted in Fig. 3c : the initial binding of a nucleotide (N) to the open binary complex (O) giving the intermediate-FRET species (IN) is described by the association constant K 1 (or its reciprocal K d1 ), whereas the conformational equilibrium between (IN) and the closed ternary complex (CN) is described by constant K 2 . In addition, the binary complex is in equilibrium between open (O) and closed (C) states, described by constant K 0 . The nucleotide titrations provide two observables ( Fig. 3a ): the first is the peak shift of the low-FRET Gaussian (comprising the unresolvable O and IN species); the halfway point, corresponding to [O]=[IN], is at a nucleotide concentration equal to K d1 . The second observable is the fraction of polymerase complexes in high-FRET conformations. We used global fitting of both observables to obtain K 0 , K 1 and K 2 ( Table 1 ). Extensions of our model are possible without altering its general conclusions; a five-state model including a potential intermediate-FRET species in the binary complex led only to a small additional scaling factor for K d1 (see Supplementary Methods ). 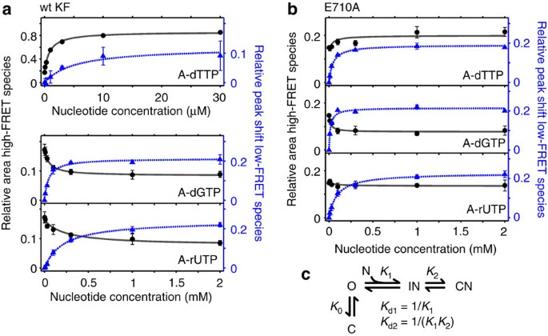Figure 3: Determining equilibrium constants for wt KF and E710A. (a,b) Nucleotide dependence of FRET observables associated with the formation of ternary complexes of wt KF (a) and E710A (b) in the presence of DNA1. The fraction of the molecules in the high-FRET species (black circles) and the shift of the meanE*of the low-FRET species (blue triangles) were plotted as a function of nucleotide concentration. The shift was normalized relative to theE*difference between the means of the open and closed conformations. Data points with error bars are represented as mean±s.e.m., derived from three independent measurements (seeSupplementary Fig. S2for examples of titrations). The data were globally fitted using a four-state equilibrium model (c). SeeTable 1for results. (c) Four-state model describing the nucleotide-concentration-dependent FRET observables (for details, see main text and Methods).K0represents the equilibrium between open and closed forms of the binary complex (O: open, C: closed). Upon nucleotide (N) addition, the nucleotide-bound intermediate-FRET state (IN) and closed state (CN) are formed sequentially. The nucleotide-dependent equilibria are described byK1andK2, respectively. The dissociation constantsKd1andKd2are calculated fromK1andK2. Figure 3: Determining equilibrium constants for wt KF and E710A. ( a , b ) Nucleotide dependence of FRET observables associated with the formation of ternary complexes of wt KF ( a ) and E710A ( b ) in the presence of DNA1. The fraction of the molecules in the high-FRET species (black circles) and the shift of the mean E* of the low-FRET species (blue triangles) were plotted as a function of nucleotide concentration. The shift was normalized relative to the E* difference between the means of the open and closed conformations. Data points with error bars are represented as mean±s.e.m., derived from three independent measurements (see Supplementary Fig. S2 for examples of titrations). The data were globally fitted using a four-state equilibrium model ( c ). See Table 1 for results. ( c ) Four-state model describing the nucleotide-concentration-dependent FRET observables (for details, see main text and Methods). K 0 represents the equilibrium between open and closed forms of the binary complex (O: open, C: closed). Upon nucleotide (N) addition, the nucleotide-bound intermediate-FRET state (IN) and closed state (CN) are formed sequentially. The nucleotide-dependent equilibria are described by K 1 and K 2 , respectively. The dissociation constants K d1 and K d2 are calculated from K 1 and K 2 . Full size image Table 1 Equilibrium constants for nucleotide binding. * Full size table With wt KF, the complementary dNTP (A-dTTP) forms the intermediate-FRET species with a K d1 of 5.1 μM ( Table 1 ); the favourable equilibrium towards the closed complex ( K 2 =6.1) augments the binding affinity so that the closed conformation is stabilized (dissociation constant of the closed ternary complex, K d2 =1/( K 1 K 2 )=0.83 μM). The affinity of incorrect nucleotides or complementary rNTPs for the intermediate state is weaker ( K d1 : 46 μM for A-dGTP, 210 μM for A-rUTP and 30 μM for A-rGTP; Table 1 ) and the low values of K 2 (<0.2 in all cases) inhibit full fingers-closing. Titrations of wt KF with nucleotides in the absence of DNA ( Supplementary Fig. S2e ) show formation of an intermediate-FRET species, as reported previously [7] . The initial binding affinity K d1 (3.0 μM for dGTP; 12 μM for rGTP) is similar to that for a correctly paired A-dTTP ternary complex; however, the subsequent transition to the closed complex is not favoured ( K 2 <0.2, Table 1 ). The conformations of wt KF with complementary and mispaired dNTPs at a template G and a template T ( Fig. 4a ) were similar to those for template A ( Fig. 2a ). 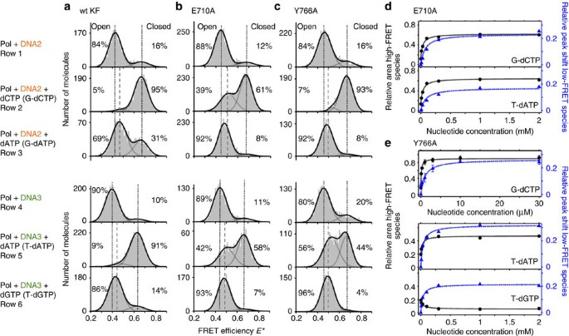Figure 4: Conformational profiles depend on the templating base. (a–c) FRET histograms for binary and ternary complexes formed using wt KF (a), E710A (b) and Y766A (c). Conditions and style are as inFig. 2, except that the DNA substrates were DNA2 (template G) or DNA3 (template T); for sequences, seeFig. 1d. (d,e) Nucleotide-concentration dependence of the conformational distribution of the E710A ternary complex with G-dCTP and T-dATP base pairs (d) and of the Y766A ternary complex with G-dCTP, T-dATP and T-dGTP base pairs (e). Data analysis was as inFig. 3; the results are shown inTable 1. Ine, the error bars on the G-dCTP plot represent the s.e. from two independent titrations; all other titrations represent single measurements. Figure 4: Conformational profiles depend on the templating base. ( a – c ) FRET histograms for binary and ternary complexes formed using wt KF ( a ), E710A ( b ) and Y766A ( c ). Conditions and style are as in Fig. 2 , except that the DNA substrates were DNA2 (template G) or DNA3 (template T); for sequences, see Fig. 1d . ( d , e ) Nucleotide-concentration dependence of the conformational distribution of the E710A ternary complex with G-dCTP and T-dATP base pairs ( d ) and of the Y766A ternary complex with G-dCTP, T-dATP and T-dGTP base pairs ( e ). Data analysis was as in Fig. 3 ; the results are shown in Table 1 . In e , the error bars on the G-dCTP plot represent the s.e. from two independent titrations; all other titrations represent single measurements. Full size image E710 has a critical role in the fingers-closing transition The conformational profiles of unliganded E710A and its binary complex with DNA1 resemble those of wt KF ( Fig. 2b , rows 1 and 2). However, addition of the complementary nucleotide (A-dTTP; Fig. 2b , row 3), even at high concentrations (≥1 mM), led to only a modest increase in the occupancy of the closed state. Instead, the bulk of the population shifted from the open state ( E* ~0.44) to an intermediate-FRET species ( E* ~0.48). The K d1 for the E710A A-dTTP ternary complex was 43 μM ( Table 1 and Fig. 3b ), similar to that for wt KF with a mispair (A-dGTP), but several fold higher than that for wt KF with the complementary A-dTTP. Further, the K 2 for the E710A A-dTTP ternary complex was <1, similar to mispairs with wt KF ( Table 1 ), preventing efficient formation of the closed conformation. The interactions of E710A with both a non-complementary dNTP (A-dGTP) and a complementary rNTP (A-rUTP) showed the same shift towards the E* ~0.48 state as with wt KF ( Fig. 2b ). With A as the templating base, E710A binds the incorrect dGTP 3-fold more tightly ( K d1 =16 μM) than does wt KF ( K d1 =46 μM); interestingly, this incorrect interaction is also threefold tighter than the binding of the correct dNTP (A-dTTP) by E710A. For the complementary rNTP (A-rUTP), both K d1 and K 2 are ~2-fold more favourable for E710A than for wt KF, probably owing to easier accommodation of the ribose 2′-OH when the glutamate side chain is replaced by alanine. The behaviour of E710A at template G and template T ( Fig. 4b ) was as described for template A, except in the presence of complementary dNTPs. Despite weak initial binding of the complementary dNTPs, the more favourable K 2 values of ~2 resulted in greater occupancy of the closed conformation (61% for G-dCTP and 58% for T-dATP at 1 mM dNTP); however, the overall affinity of E710A for all three complementary base pairs is low ( Fig. 4d , Table 1 ), indicating that E710A discriminates poorly between correct and mispaired dNTPs regardless of templating base. The conformational profile for E710Q at template A ( Fig. 2d ) was similar to that of E710A ( Table 1 ). Y766A perturbs fingers-closing for complementary dNTPs With template bases A and T, the Y766A mutator followed the pattern seen for E710A and E710Q ( Figs 2d and 4c ). Addition of complementary nucleotides (A-dTTP or T-dATP) led to equal occupancy of the intermediate-FRET and high-FRET states at high nucleotide concentrations (≥1 mM). Addition of incorrect nucleotides (A-dGTP, G-dATP, or T-dGTP) formed predominantly the intermediate-FRET species. At template A and T, all dNTPs showed weak binding regardless of their complementarity to the templating base ( Table 1 ). However, at template G, Y766A bound the complementary dCTP as strongly as wt KF ( K d1 =1.0 μM for Y766A versus 1.2 μM for wt KF, Fig. 4e ) and formed the closed complex almost exclusively, reflecting a very favourable K 2 ( Table 1 ). Moreover, the single-turnover kinetic parameters for G-dCTP incorporation by Y766A and wt KF ( Supplementary Table S2 ) are similar, in contrast to those for A-dTTP incorporation. Thus, at template G, Y766A distinguishes well between correct and incorrect dNTPs. The complexes of Y766F, which has similar fidelity to wt KF [11] , [14] , resembled those of wt KF ( Fig. 2e , Table 1 ), the only difference being a ~3-fold decreased binding affinity ( K d1 ) for the complementary nucleotide (A-dTTP) and an increased K 2 (9.6) so that the overall K d2 is ~2-fold weaker for Y766F. Y766 modulates the equilibrium in unliganded polymerases Whereas the unliganded wt KF, E710A and E710Q polymerases exhibit similar conformational equilibria, Y766 substitutions shift the equilibrium ( Fig. 2d ). Loss of the bulky phenyl ring from the Y766 side chain increases the open-state occupancy to 78% (Y766A), whereas the more conservative Y766F substitution, which removes a potential hydrogen-bond donor, decreases the open-state occupancy to 28%. The large differences between wt KF, Y766A and Y766F indicate that the interconversion rates between open and closed states depend on residue 766. To characterize the equilibria, we used probability distribution analysis (PDA) [8] , [17] , [18] and burst variance analysis (BVA) [7] , [10] , both described in Methods. PDA revealed that the FRET distribution fits well either to a ‘static’ model of two independent molecular entities or a ‘dynamic’ model [19] , [20] that invokes dynamic interconversions of a single molecular entity between two distinct FRET states ( Fig. 5a , top). 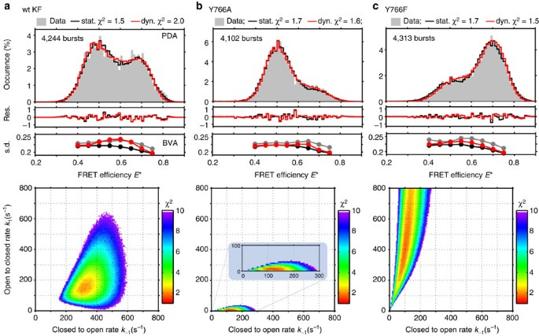Figure 5: Conformational dynamics of unliganded wt KF and Y766 derivatives. (a) Analysis of wt KF using PDA (upper panel), BVA (middle panel) and a rate-dependent PDAχ2-minimization surface (lower panel). TheE*histogram was fitted using PDA, assuming either a static (black line) or a dynamic (red line) two-species model, wherein the polymerase occupies either the closed or open state yieldingk1=150 s−1, andk−1=320 s−1for the dynamic model (seeSupplementary Methodsfor fitting parameters). Whereas PDA achieved satisfactory fits to the data in either scenario, as shown by the residuals plot (χ2≤2), the BVA data (grey line) favoured the dynamic model (red line). The PDAχ2-minimization surface uses the mean FRET positions and excess widths from the dynamic fit, plotting theχ2<10 values as a function of the rates. Best fits are obtained fork1~160 s−1andk−1~320 s−1. (b,c) Analysis of conformational dynamics for Y766A and Y766F, as ina, yielding interconversion rates ofk1=9 s−1,k−1=128 s−1for Y766A andk1=435 s−1, andk−1=108 s−1for Y766F. For fitting parameters, seeSupplementary Methods; for PDA of the wt KF binary complex and the wt KF ternary complex with an incorrect nucleotide, seeSupplementary Fig. S4. Figure 5: Conformational dynamics of unliganded wt KF and Y766 derivatives. ( a ) Analysis of wt KF using PDA (upper panel), BVA (middle panel) and a rate-dependent PDA χ 2 -minimization surface (lower panel). The E* histogram was fitted using PDA, assuming either a static (black line) or a dynamic (red line) two-species model, wherein the polymerase occupies either the closed or open state yielding k 1 =150 s −1 , and k −1 =320 s −1 for the dynamic model (see Supplementary Methods for fitting parameters). Whereas PDA achieved satisfactory fits to the data in either scenario, as shown by the residuals plot ( χ 2 ≤2), the BVA data (grey line) favoured the dynamic model (red line). The PDA χ 2 -minimization surface uses the mean FRET positions and excess widths from the dynamic fit, plotting the χ 2 <10 values as a function of the rates. Best fits are obtained for k 1 ~160 s −1 and k −1 ~320 s −1 . ( b , c ) Analysis of conformational dynamics for Y766A and Y766F, as in a , yielding interconversion rates of k 1 =9 s −1 , k −1 =128 s −1 for Y766A and k 1 =435 s −1 , and k −1 =108 s −1 for Y766F. For fitting parameters, see Supplementary Methods ; for PDA of the wt KF binary complex and the wt KF ternary complex with an incorrect nucleotide, see Supplementary Fig. S4 . Full size image We used BVA to show that the dynamic model prediction fitted the data significantly better than the static model ( Fig. 5a ), suggesting the presence of dynamic heterogeneity for all three KF derivatives. To further analyse the conformational dynamics, we performed PDA using the FRET efficiencies E* i obtained from the initial PDA fit (dynamic model), and plotted the χ 2 -values as a function of k 1 and k −1 ( Fig. 5a , bottom). For wt KF, the minimization surface forms a distinct well at k 1 =160 s −1 and k −1 =320 s −1 ( χ 2 <2), consistent with our previous reports [7] , [8] , [10] . In contrast, both Y766A and Y766F display different landscapes ( Figs. 5b ), whereas Y766A shows a distinct well at k 1 =15 s −1 and k −1 =120 s −1 , Y766F displays a broad range of possible rate combinations with a shallow minimum at k 1 ~450 s −1 and k −1 ~120 s −1 . Accessing the equilibrium dynamics of wt KF complexes To characterize the timescales of interconversions within the sequential four-state model ( Fig. 3c ), we used PDA and a novel analysis of FRET distribution widths. Using PDA, we characterized the interconversions between O and C for the wt KF binary complex, and between IN and CN for the wt KF ternary complex with an A-dGTP mispair at saturating nucleotide conditions ( Supplementary Fig. S4 ); this analysis yielded rate constants of k O→C =15 s −1 and k C→O =85 s −1 for the binary complex and k IN→CN =3 s −1 and k CN→IN =45 s −1 for the mispaired ternary complex. Accessing the remaining rates (corresponding to rate constants k O→IN and k IN→O ) is challenging, as the analysis of the low-FRET species is hampered by our inability to resolve the FRET distributions of the O and IN states. Width analysis (see Methods) of our data ( Supplementary Fig. S5c ) revealed broadening of the low-FRET species around K d1 for several nucleotide titrations (for wt KF: A-dGTP and A-rUTP; for E710A: A-dTTP, A-dGTP and A-rUTP), indicating that the interconversions are at the millisecond timescale or slower. For the E710A A-rUTP titrations, for example, there is a maximum broadening of ~6% at 100 μM rUTP, close to the corresponding K d1 of 92 μM. For a better estimate of the timescale, we simulated the four-state model using four fixed rates (by fixing k O→C , k C→O , k IN→CN and k CN→IN ) and varying k O→IN and k IN→O ( Supplementary Fig. S5d ; as in Santoso et al . [7] ). The width of the low-FRET species at a nucleotide concentration equal to K d1 remains constant for high IN-to-O rates (≥300 s −1 ), whereas for rates of <300 s −1 there is a significant width increase around K d1 . We thus propose a rate of 300 s −1 as an upper limit for the IN-to-O transition. Previously, we described a FRET state between the open and closed states for wt KF ternary complexes with incorrect nucleotides [7] . Data presented here strongly suggest that wt KF accesses this intermediate state even with complementary dNTPs, consistent with this state being on the path to nucleotide incorporation. Whereas the intermediate-FRET state is sparsely populated in the ternary complex of wt KF with a complementary dNTP, the three mutators (Y766A, E710A and E710Q) behave differently; their ternary complexes with complementary dNTPs occupy mainly the intermediate-FRET state, with Y766A and the G-dCTP base pair being the only exception. Initially, we attempted to relate the intermediate-FRET species to available cocrystal structures, speculating that the ternary complex with a complementary rNTP undergoes partial fingers closure, whereas the mispaired ternary complex resembles a fingers-open conformation [7] . Since then, a better structural candidate for the intermediate-FRET species has been described [21] . Using Bacillus stearothermophilus DNA polymerase (a KF homologue), Wu and Beese [21] captured a partially closed (‘ajar’) fingers conformation ( Fig. 6a ) in a ternary complex with a G-dTTP mismatch, using both a mutator (Y714S, equivalent to Y766S in KF) and a non-mutator (F710Y, equivalent to F762Y in KF) polymerase; the partially closed state corresponds to fingers-closing along the open-to-closed transition, leading to a distance change of ~2 Å between the sites carrying the FRET probes, in excellent agreement with our observations. 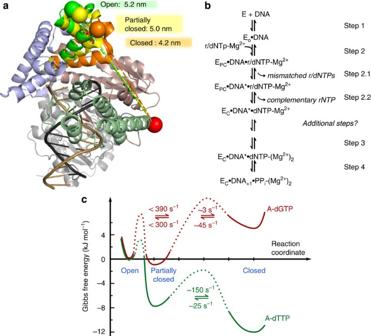Figure 6: Roles of the partially closed state in nucleotide selection. (a) Proposed structure of the polymerase conformation corresponding to the intermediate-FRET state. The crystal structure of the Pol-DNA binary complex (PDB accession code1L3U, mobile section green)4is superimposed on the crystal structures of a ternary complex where the fingers adopt a partially closed (‘ajar’) conformation (PDB accession code3HPO, mobile section yellow)21and a ternary complex where the fingers adopt the closed conformation (PDB accession code1LV5, mobile section orange)4. The distances between the Cβpositions of residue 550 (red sphere on the thumb) and 744 (sphere on the fingers) are 5.2 nm in the open, 5.0 nm in the partially closed and 4.2 nm in the closed conformation. The predicted distance change of ~2 Å on going from the open to the partially closed conformation is consistent with the observed shift of ΔE*~0.04, as we operate in the linear part of the FRET dynamic range. (b) Proposed reaction pathway for KF from DNA binding to phosphoryl transfer, based on references7,21,23and our current results. EOand ECrepresent the open and the closed conformations, respectively, whereas EPCrepresents the intermediate-FRET state interpreted as a partially closed conformation. (c) Proposed free-energy landscapes for the prechemistry nucleotide selection steps prepared using the equilibrium constants inTable 1andin vivodNTP concentrations27(green curve: complementary nucleotide A-dTTP; red curve: non-complementary nucleotide A-dGTP; see also Methods). Reaction coordinate: degree of fingers-closing (shown to scale). The free energy of the open binary state is set to zero. Binding of a nucleotide stabilizes the complex with the partially closed conformation, either weakly (incorrect base pair A-dGTP) or strongly (correct base pair A-dTTP). Equilibration to the fully closed conformation is favoured only for the correct nucleotide. Although the exact activation energy barriers (dotted lines) between the conformations are unknown, we included the rates for the transition of the A-dGTP ternary complex between the open and partially closed states (estimated using FRET-width analysis;Supplementary Fig. S5) and the rates for the transitions between the partially closed and the closed states for correct and incorrect nucleotides (determined using PDA;Supplementary Figs S1c and S4, respectively). Figure 6: Roles of the partially closed state in nucleotide selection. ( a ) Proposed structure of the polymerase conformation corresponding to the intermediate-FRET state. The crystal structure of the Pol-DNA binary complex (PDB accession code 1L3U , mobile section green) [4] is superimposed on the crystal structures of a ternary complex where the fingers adopt a partially closed (‘ajar’) conformation (PDB accession code 3HPO , mobile section yellow) [21] and a ternary complex where the fingers adopt the closed conformation (PDB accession code 1LV5 , mobile section orange) [4] . The distances between the C β positions of residue 550 (red sphere on the thumb) and 744 (sphere on the fingers) are 5.2 nm in the open, 5.0 nm in the partially closed and 4.2 nm in the closed conformation. The predicted distance change of ~2 Å on going from the open to the partially closed conformation is consistent with the observed shift of Δ E* ~0.04, as we operate in the linear part of the FRET dynamic range. ( b ) Proposed reaction pathway for KF from DNA binding to phosphoryl transfer, based on references [7] , [21] , [23] and our current results. E O and E C represent the open and the closed conformations, respectively, whereas E PC represents the intermediate-FRET state interpreted as a partially closed conformation. ( c ) Proposed free-energy landscapes for the prechemistry nucleotide selection steps prepared using the equilibrium constants in Table 1 and in vivo dNTP concentrations [27] (green curve: complementary nucleotide A-dTTP; red curve: non-complementary nucleotide A-dGTP; see also Methods). Reaction coordinate: degree of fingers-closing (shown to scale). The free energy of the open binary state is set to zero. Binding of a nucleotide stabilizes the complex with the partially closed conformation, either weakly (incorrect base pair A-dGTP) or strongly (correct base pair A-dTTP). Equilibration to the fully closed conformation is favoured only for the correct nucleotide. Although the exact activation energy barriers (dotted lines) between the conformations are unknown, we included the rates for the transition of the A-dGTP ternary complex between the open and partially closed states (estimated using FRET-width analysis; Supplementary Fig. S5 ) and the rates for the transitions between the partially closed and the closed states for correct and incorrect nucleotides (determined using PDA; Supplementary Figs S1c and S4 , respectively). Full size image Evidence for a partially closed state was also reported in a recent FRET study on immobilized KF complexes [22] . In contrast to our assay, which reports directly on conformational states by monitoring an intra-protein distance, Berezhna et al . [22] used donor-labelled DNA and acceptor-labelled polymerases to infer a protein conformational change by measuring a DNA-protein distance; in the latter assay, any protein conformational changes may be superimposed on concurrent DNA conformational changes, as well as on possible polymerase repositioning relative to the DNA. The partially closed cocrystal structures may also relate to other intermediate-FRET species we have observed. By introducing a mutation that prevents full closing of the O-helix, Wu and Beese [21] captured a partially closed B. stearothermophilus ternary complex with a correctly paired dNTP, a candidate for the sparsely populated species of intermediate-FRET value in the ternary complexes of wt KF with correct dNTPs. More speculatively, we note that the Pol-dNTP binary complex (without DNA) has a similar intermediate-FRET signature ( Supplementary Fig. S2e ; see also Santoso et al . [7] ), suggesting that O-helix movement might be initiated by dNTP binding in the KF cleft without direct DNA involvement. Our K d measurements ( Table 1 ) indicate that nucleotide binding is destabilized by the presence of DNA with a non-complementary template base, just as DNA binding is destabilized by a mismatched dNTP (O.B., N.D.F.G., C.M.J, unpublished) [23] ; both cases promote dissociation of mispaired ternary complexes. It seems reasonable to assume that the partially closed complex is on the pathway to the chemical step, given that the partially closed state is structurally part way between open and closed states. We cannot directly rule out the alternative scenario whereby the partially closed conformation is an ‘off-pathway’ state in equilibrium with the open but not the closed state as, in either case, the equilibria follow similar relations ( Supplementary Methods ). The partially closed conformation has the hallmarks of an early checkpoint, being populated in all wt KF ternary complex species, although these species progress differently along the reaction pathway. This conformation must be formed at an early step, most probably immediately after the Pol-DNA binary complex binds a nucleotide and its Mg 2+ ion (step 2, Fig. 6b ). Although our FRET pair does not distinguish between mispaired and rNTP-containing ternary complexes, experiments using 2-aminopurine on DNA substrates show that wt KF complexes with a complementary rNTP proceed further than mispairs (O.B., N.D.F.G., C.M.J, unpublished) [23] . A nanopore-based study of single KF–DNA complexes also supports this conclusion [24] . The partially closed conformation, therefore, encompasses at least two related ternary complexes ( Fig. 6b ) whose equilibria determine the progression of a particular ternary complex towards product formation. First, the partially closed ternary complex undergoes a base-checking step (step 2.1) in which the equilibrium is unfavourable for all non-complementary nucleotides (dNTPs and rNTPs), thus rejecting six out of the eight nucleoside triphosphates. Next, the sugar structure is tested against the active-site pocket (step 2.2), rejecting the bulkier rNTPs and allowing complexes containing complementary dNTPs to proceed to the closed conformation, from which they undergo subsequent steps, including D705 reorientation and binding of the second Mg 2+ ion [25] . The calculated equilibrium constants ( Table 1 ) enabled us to propose a free-energy landscape for the prechemistry nucleotide selection steps ( Fig. 6c ). Although a simplified landscape has been proposed before (on the basis of fluorescence enhancement of a dye-labelled DNA upon T7 DNA polymerase binding [26] ), our ability to monitor the conformational coordinate directly allowed us to add the important partially closed conformation checkpoint. The dissociation constant for a nucleotide in the partially closed ternary complex, K d1 , reports on interactions in the wt KF active site. The binding of the complementary dNTP is favoured, leading to a stabilized partially closed state (−8 kJ mol −1 for A-dTTP versus −0.7 kJ mol −1 for A-dGTP, using the nucleotide concentrations in E. coli [27] ); this may result from tighter binding within either or both of E PC ·DNA·r/dNTP-Mg 2+ and E PC ·DNA*·r/dNTP-Mg 2+ (see Fig. 6b ). Moreover, the similar K d1 values for A-dGTP and A-rGTP complexes ( Table 1 ) indicate that the ribose 2'-OH is not detected in the initial E PC ·DNA·r/dNTP-Mg 2+ complex. K 2 , describing the equilibrium between partially closed and closed complexes, defines the free energy of the closed ternary complex. When K 2 is >1, as for correctly paired ternary complexes of wt KF, the closed complex is the lowest-energy species (−4 kJ mol −1 relative to the A-dTTP partially closed state) on the prechemistry pathway, and its enhanced stability relative to the partially closed ternary complex ( K d2 < K d1 ) drives the forward reaction. With an inappropriate substrate, such as a mispair, K 2 is <1 so that the closed complex is destabilized relative to the partially closed ternary complex (+6 kJ mol −1 for A-dGTP) and the equilibrium favours species formed early in the pathway. The extremely slow rates for misinsertion (≥10 3 -fold slower than complementary dNTP additions) probably result from low occupancy of the closed conformation combined with active-site distortions [13] , [14] . The fidelity mutants in this study show a reduced ability to recognize complementary dNTPs as ‘correct’ ( Table 1 ), having lower affinity for the initial binding of the complementary dNTP to the partially closed complex and an unfavourable K 2 . Therefore, the partially closed conformation is highly populated in the resulting ternary complexes so that, in the absence of the E710 or Y766 side chains, the complex with the complementary dNTP resembles a mispaired complex. Our data show a continuum of behaviours, with both the templating base and the particular mutator allele influencing how far the conformational equilibria shift towards the closed state; at one extreme is the E710A A-dTTP complex, which has little of the closed conformation ( K 2 =0.25), at the other is the Y766A G-dCTP complex, which resembles wt KF ( K 2 =8.9); in between are several complexes with K 2 ~1, having substantial amounts of both closed and partially closed complexes. Why should alteration of E710 or Y766 destabilize the closed ternary complex? Structurally, E710 and Y766 define much of the surface of the active site-binding pocket so that they interact more closely with the nascent base pair in the closed complex than in the partially closed complex, where the base pair is more solvent exposed. Surprisingly, the hydrogen bond between E710 and Y766, despite being invariant in A-family DNA polymerases, has a minor role in the closed complex stability, as shown by the similar FRET profile for complexes of Y766F and wt KF. More important may be the overall size and shape of the 766 side chain and its ability to interact with and position the nearby F762 side chain, which forms part of the binding pocket. Structural studies argue that the transition from partially closed to fully closed conformation is required for catalysis of the polymerase reaction. In the partially closed conformation, the primer 3′-OH is too far from the α-phosphate of the bound nucleotide; moreover, the rest of the active site, including the catalytic metal ions, is not properly assembled for a chemical attack [21] . Our data support this reasoning, showing a rough correlation between the rate of nucleotide incorporation ( k pol , Supplementary Table S2 ) and closed-complex occupancy; the most notable example is G-dCTP incorporation by Y766A, where high occupancy of the closed complex correlates with near-wild-type kinetics. Moreover, for the mutator proteins, the single-turnover K d for A-dTTP incorporation ( K d(dNTP) , Supplementary Table S2 ) approximates to K d2 ( Table 1 ), consistent with closed-complex formation being required for the chemical step. (This assumes that the chemical step is rate limiting for these mutant proteins. For wt KF (and probably Y766F), the same relationship does not hold, as prechemistry step 3 is rate limiting) [28] . Nevertheless, as the low incorporation rate for E710Q shows ( Supplementary Table S2 ), achieving the closed state with moderate efficiency is, of itself, no guarantee of effective catalysis if the mutation distorts the final active-site geometry. Our data support the generalization that alterations in polymerase fidelity correlate with the kinetics of handling correct, rather than incorrect, nucleotides [29] . Compared with wt KF, the mutator variants show at most a threefold enhancement in the binding ( K d1 ) of the non-complementary A-dGTP and no improvement in K 2 . This contrasts with the much larger deficits in both constants for the mutators when binding the correct A-dTTP. As the closed complex selects for the correct template-dNTP pairing, any change to the energetics of this complex will exclusively affect correct dNTP incorporation. Moreover, even in the partially closed conformation, changes in active-site side chains diminish specificity for the correct pairing more than they enhance the interaction with mispairs. The effects of template base and mutator allele on closed-complex energetics provide a partial explanation of the observed error specificities of the KF mutators ( Supplementary Fig. S6 ) [11] , [12] , [13] , [14] . Closed complexes with the correct dNTP are least populated when E710A encounters template A or when Y766A encounters template A or T, making these the situations where recognition of the correct base pair is least effective. One would therefore expect E710A to be less accurate at template A than that at G or T, and Y766A to be less accurate at templates A and T, relative to G. This is consistent with the high frequency of A-dCTP errors made by E710A and T-dGTP made by Y766A but does not explain the lower frequency of other errors at these particular template bases. The substantial frequency of Y766A G-dTTP errors is noteworthy, given that Y766A handles the G-dCTP pair with almost wild-type efficiency; this could be a case where a mutator actually facilitates the interaction with the mispair, consistent with earlier kinetic data [14] . As the experimentally observed polymerase errors in Supplementary Fig. S6 require not only covalent addition of mispaired bases but also extension of the resulting mismatched primer termini, they will be influenced by steric or geometric constraints in intermediates for both reactions so that the overall error specificity reflects the combination of several factors. Finally, our results on the unliganded Y766 polymerase derivatives reinforce our previous observations that the conformational equilibrium of the unliganded polymerase is delicate; thus, the removal of even a single oxygen atom (as in Y766F) increased substantially the occupancy of the closed state for the unliganded polymerase, whereas the more drastic Y766A mutation had the opposite effect. By contrast, changes to the 710 side chain did not influence the conformational equilibrium, suggesting that the behaviour of Y766 derivatives is not directly related to the missing 710–766 hydrogen bond in the closed conformation. An alternative explanation considers, instead, the open conformation, where the 766 side chain is extremely solvent exposed; one might expect the side chains to favour the open conformation in the reverse order of their hydrophobicity: A>Y>F, as is observed. Unlike the unliganded polymerase, the FRET distributions of binary complexes of the mutant and wt polymerases were similar, indicating that the conformational landscape is dominated by Pol-DNA interactions, and that the apparent conformational equilibrium of unliganded polymerases is not a reliable predictor of the conformational landscape of the corresponding binary complexes. Single-molecule FRET measurements Single-molecule FRET experiments were performed at room temperature (≈22 °C) using a home-built confocal microscope equipped with 20 kHz alternating laser excitation between a 532-nm (operated at 240 μW) and a 638-nm laser (operated at 60 μW), coupled to a × 60, 1.35 NA, UPLSAPO 60XO (Olympus) objective. The alternating laser excitation allows filtering for correctly labelled species bearing an active donor and an active acceptor [30] . After filtering each fluorescent burst for the correct labelling stoichiometry, we calculated the apparent FRET efficiency E* for each burst as E* =DA/(DD+DA), where DA is the number of photons in the red detection channel after green excitation and DD the number of photons in green detection channel after green excitation. Doubly labelled KF derivatives were present at <100 pM in single-molecule observation buffer (40 mM 4-(2-hydroxyethyl)-1-piperazineethanesulfonic acid (HEPES)-NaOH, pH 7.3, 10 mM MgCl 2 , 1 mM dithiothreitol, 100 μg ml −1 bovine serum albumin, 5% (vol/vol) glycerol, 1 mM mercaptoethylamine). Analysis of FRET histograms Single-molecule FRET experiments are sensitive to subtle changes in conditions such as room temperature and set-up alignment [30] , [31] . To minimize changes, every set of experiments contains reference measurements of a DNA FRET standard with a reference FRET value of E *~0.5 (ref. 32 ), the unliganded polymerase, the binary complex formed with DNA and the ternary complex with DNA and nucleotides. Each titration experiment was completed in a single day. The stoichiometry-filtered E * FRET histograms were fitted to double-Gaussian functions that were constrained by a maximum width of σ max ( E *)≤0.07. The double Gaussians report on peak positions and relative occupancies. For titration experiments, we plotted the relative peak shift ( E* obs − E* open )/( E* closed − E* open ) of the low-FRET Gaussian and the fractional occupancy of the high-FRET Gaussian as a function of nucleotide concentration. We fixed the position of the high-FRET Gaussians to the value obtained from a free fit of the binary complex or a saturated ternary complex with complementary dNTPs. We did not fix the position of the low-FRET Gaussian. Derivation of the multistate equilibrium model To determine the parameters governing the equilibria between the species observed in the single-molecule FRET histograms ( Fig. 3c ), we derived equations for the two concentration-dependent FRET observables: the peak position of the low-FRET Gaussian and the fraction of the population in the high-FRET Gaussian. The binary complex is in dynamic equilibrium between open (O, low-FRET) and closed (C, high-FRET) conformations, described by the equilibrium constant K 0 =[C]/[O]. Binding of a nucleotide (N) to the open conformation, forming the intermediate-FRET ternary complex (IN), is described by the association constant K 1 =[IN]/[O][N]. The intermediate-FRET ternary complex can undergo an additional conformational transition to the closed ternary complex (CN, high-FRET), governed by the equilibrium constant K 2 =[CN]/[IN]. The corresponding dissociation constants are defined as K d1 =1/ K 1 for the formation of the intermediate-FRET state and K d2 =1/( K 1 K 2 ) for the formation of the high-FRET (fully closed) state. The total polymerase concentration is The fractions of each species as a function of nucleotide concentration are: The two FRET observables are given (a) by the normalized peak shift of the low-FRET Gaussian where y max corresponds to the normalized peak shift at saturating nucleotide concentration and (b) by the fraction of high-FRET species We used a global fitting approach to fit both FRET observables simultaneously as a function of nucleotide concentration, and to determine the equilibrium constants K 0 , K 1 and K 2 , and the parameter y max . From the equilibrium constants and their s.e., we calculated the dissociation constants. Identical equations can be derived to describe nucleotide binding to the polymerase in the absence of DNA; in this case, O and C refer to the unliganded protein. Probability distribution analysis and burst variance analysis For PDA [8] , the static model is fully described by two peak positions E* i , two excess widths σ i (accounting for additional broadening of <E* i > due to acceptor photophysics [17] , [19] ) and two relative occupancies N i . In comparison, the dynamic model replaces the relative occupancies with two rate constants: k 1 for the open-to-closed transition and k −1 for the closed-to-open transition. We optimized parameters for both models using a least mean square algorithm implemented in MATLAB. BVA directly evaluates FRET distributions for the presence of dynamic heterogeneity [10] . In BVA, the experimentally measured s.d. of the FRET efficiency for individual transits through the confocal spot is compared with the s.d. predicted by the static and dynamic models. Width analysis for obtaining rate constants At nucleotide concentrations equal to the dissociation constant K d1 (where [O] equals [IN]), the interconversion rates between O and IN, k O→IN and k IN→O , are equal. These rates also control the width of the low-FRET species distribution: if k O→IN and k IN→O are high and lead to multiple interconversions during the transit of the complex through the detection volume (~3 ms (ref. 7 )), the FRET averaging between O and IN will yield a FRET width for the low-FRET species that matches that for the binary or partially closed ternary complex for all nucleotide concentrations. In contrast, slower interconversions will lead to a FRET-width increase; this increase should peak around K d1 ( Supplementary Fig. S5a,b ). Calculating the free-energy landscape of ternary complexes To construct the free-energy landscape for the prechemistry conformations of wild-type DNA polymerase in the presence of nucleotides, we calculated the relative Gibbs free energies Δ r G for the partially closed conformation and the fully closed conformation in ternary complexes by using the open conformation in the binary complex as a reference. To estimate Δ r G (O/IN) , the free-energy difference between the open conformation and the partially closed conformation, for a complementary dNTP (A-dTTP), we used: Δ r G =Δ r G 0 + RT ln( Q r ). The first term, Δ r G 0 , is the free energy corresponding an O-to-IN equilibrium with 1 M concentrations for all species involved and is calculated using Δ r G 0 =− RT ln( K 1 ), where R is the ideal gas constant, T the temperature and K 1 is the equilibrium association constant measured using our nucleotide titration experiments ( Table 1 ). The second term requires the reaction quotient Q r , which is a function of the actual concentrations of all species involved in the equilibrium: Q r ={[IN]/[O][N]}. To estimate Q r , we set [N] to the E.coli intracellular concentration for dTTP (120 μM) [27] , and assumed that [IN]=[O]. To estimate Δ r G (IN/CN) , the free-energy difference between the partially closed conformation and the closed conformation with bound nucleotide, we used Δ r G (IN/CN) =− RT ln( K 2 ). Similar expressions were used for the free energies of the ternary complexes formed upon binding to an incorrect dNTP (A-dGTP); for dGTP, we used [N]=60 μM [27] . Using the proposed rate of ~300 s −1 as an upper limit for the rate of the IN-to-O transition for A-dGTP, we calculate the rate of the O-to-IN transition at 60 μM dGTP in E.coli as follows: rate= K 1 · k IN→O · 60 μM=21.7·10 3 M −1 · 300 s −1 · 60·10 −6 M=390 s −1 . The following procedures are further described in the Supplementary Methods : DNA preparation, protein expression and purification, and site-specific labelling of KF. How to cite this article: Hohlbein, J. et al. Conformational landscapes of DNA polymerase I and mutator derivatives establish fidelity checkpoints for nucleotide insertion. Nat. Commun. 4:2131 doi: 10.1038/ncomms3131 (2013).